Cell wall elongation mode in Gram-negative bacteria is determined by peptidoglycan architecture Cellular integrity and morphology of most bacteria is maintained by cell wall peptidoglycan, the target of antibiotics essential in modern healthcare. It consists of glycan strands, cross-linked by peptides, whose arrangement determines cell shape, prevents lysis due to turgor pressure and yet remains dynamic to allow insertion of new material, and hence growth. The cellular architecture and insertion pattern of peptidoglycan have remained elusive. Here we determine the peptidoglycan architecture and dynamics during growth in rod-shaped Gram-negative bacteria. Peptidoglycan is made up of circumferentially oriented bands of material interspersed with a more porous network. Super-resolution fluorescence microscopy reveals an unexpected discontinuous, patchy synthesis pattern. We present a consolidated model of growth via architecture-regulated insertion, where we propose only the more porous regions of the peptidoglycan network that are permissive for synthesis. Peptidoglycan is the main stress-bearing component of the bacterial cell wall [1] , [2] , [3] . In cylindrical Gram-negative bacteria, glycan chains are currently thought to run roughly circumferentially around the cell in a single layer [4] . These have been hypothesized to be organized in tessera, hexagonal regions bounded by two non-asaccharides and two peptide cross bridges, where alternate peptides participate in cross-bridges [5] . Glycan strands have a theoretically higher spring constant than the peptides enabling them to resist the circumferential hoop stress, which is twice the longitudinal stress when the cell is modelled as a thin-walled pressure vessel [6] . This would allow cylindrical shape to be maintained, and is the basis of more sophisticated numerical models [7] . Peptidoglycan architecture must be propagated accurately for the cell to grow. This requires that new peptidoglycan is inserted in a way that maintains the integrity, shape and thickness of the existing sacculus, whereas continually resisting turgor pressure. Although the peptidoglycan insertion pattern is quite well established in Gram-positive organisms [8] , [9] , [10] , [11] , there has been a long running conflict between models of peptidoglycan insertion during elongation in Gram-negative bacteria [12] , including proposals of helical [13] and diffuse [14] modes. Localization of some of the proteins required for peptidoglycan synthesis, for example, Mre and Lpo proteins [15] , [16] , [17] , goes some way towards settling this matter. However, an overarching growth model requires a direct means of localizing insertion at high resolution and for this pattern to be related to peptidoglycan architecture. Here, we apply tapping mode Atomic Force Microscopy (AFM) and fluorescence microscopy that we have previously used to reveal architecture in several Gram-positive species [10] , [11] , [18] , along with super-resolution Stochastic Optical Reconstruction Microscopy (STORM) [19] , [20] to develop a new model of cell wall elongation in Gram-negative bacteria. Escherichia coli peptidoglycan architecture Gram-negative sacculi were purified using standard methods. The relatively flat profile of the Gram-negative sacculi and imaging sacculi in liquid revealed significantly more architectural detail than previous AFM studies ( Fig. 1 and Supplementary Fig. S1 ), as well as the now-familiar folds and trapped cytoplasmic material [10] , [11] , [18] , [21] . 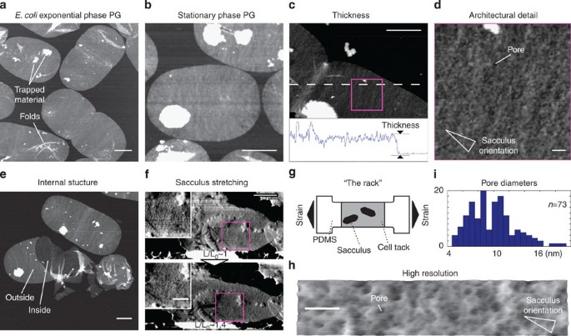Figure 1: Tapping Mode AFM images of peptidoglycan architecture inE. coliMC1061. (a) Sacculi imaged under water showing banded variation, folds and trapped cytoplasmic contents (scale bar, 500 nm; height, 10 nm). (b) Stationary-phase sacculi imaged in ambient conditions (scale bar, 500 nm; height, 5 nm). (c) Sacculus in ambient conditions; material is thicker at the septum (scale bar, 500 nm; height, 10 nm); cross-section (dotted line) shows height variation and site of thickness measurements (distance between arrows 3 nm). (d) Enlargement of boxed region: bands are made up of less-ordered “filigree” features (scale bar, 50 nm; height, 5 nm). (e) Sacculi imaged in ambient conditions showing internal and external architecture (scale bar, 500 nm; height, 7 nm). (f) Mechanical stretching (“The Rack”) of sacculus tethered to Cell Tack in ambient conditions, showing maintenance of banding under approximately × 1.4 strain (main image scale bar, 500 nm; phase, 10°; inset scale bar, 200 nm, phase, 1.6°). (g) Diagram of “The Rack”. (h) High-resolution AFM image of part of a sacculus in water rendered in a three-dimension, pitch 14° (scale bar, 50 nm). (i), Pore-size distribution fromh(n=73). Figure 1: Tapping Mode AFM images of peptidoglycan architecture in E. coli MC1061. ( a ) Sacculi imaged under water showing banded variation, folds and trapped cytoplasmic contents (scale bar, 500 nm; height, 10 nm). ( b ) Stationary-phase sacculi imaged in ambient conditions (scale bar, 500 nm; height, 5 nm). ( c ) Sacculus in ambient conditions; material is thicker at the septum (scale bar, 500 nm; height, 10 nm); cross-section (dotted line) shows height variation and site of thickness measurements (distance between arrows 3 nm). ( d ) Enlargement of boxed region: bands are made up of less-ordered “filigree” features (scale bar, 50 nm; height, 5 nm). ( e ) Sacculi imaged in ambient conditions showing internal and external architecture (scale bar, 500 nm; height, 7 nm). ( f ) Mechanical stretching (“The Rack”) of sacculus tethered to Cell Tack in ambient conditions, showing maintenance of banding under approximately × 1.4 strain (main image scale bar, 500 nm; phase, 10°; inset scale bar, 200 nm, phase, 1.6°). ( g ) Diagram of “The Rack”. ( h ) High-resolution AFM image of part of a sacculus in water rendered in a three-dimension, pitch 14° (scale bar, 50 nm). ( i ), Pore-size distribution from h ( n =73). Full size image E. coli sacculi derived from several bacterial strains, and from both exponential and stationary-phase cells, exhibited roughly circumferential light and dark bands ( Fig. 1a-e and Supplementary Fig. S1 ). AFM generates contrast from relative height, so the light bands contained more material than the dark ones. These bands were discontinuous and did not fully encircle the cells, nor had they a defined periodicity or distinct edges, and thickness varied continuously from one band to the next; band orientation was 90° (s.d. 20°, n =166), relative to the long axis of the sacculi. The thickness of the sacculi was 2.0 nm (s.d. 0.3, n =18, Fig. 1c ); mean length was 2.0 μm (s.d. 0.6, n =60) and width was 1.3 μm (s.d. 0.3, n =60). Filamentous mutant E. coli cells contract by ~17% when exposed to detergent [22] . This shrinkage could, hypothetically, introduce an artefactual concertina effect on the sacculus, leading to the observed banding. To simulate the effects of turgor pressure on the sacculi, we constructed “the rack” an apparatus that allowed us to apply strain to a sample during AFM ( Fig. 1f–g and Supplementary Movie S1 ). The banding pattern remained visible under longitudinal strain ( Fig. 1f and Supplementary Fig. S1i-k ), implying that it would also be present in an intact cell experiencing turgor pressure. The circumferentially oriented bands (tens by hundreds of nm) were too large to be glycan strands. To probe their nanoscale architecture, we carried out higher resolution AFM and found that they were made up of a porous “filigree” network ( Fig. 1h ). Crucially, this network exhibited no general orientation. However, there were instances when circumferential orientation of features was observed ( Supplementary Fig. S1f-g ). The height variation seen across intact ( Fig. 1 ) and broken ( Fig. 2a and Supplementary Figs. S1l-p ) sacculi shows that the peptidoglycan layer must be viewed as a polymer network where strands can be loosely or densely packed, and can overlap each other forming a continuum. Our data are not compatible with the tessera model of peptidoglycan architecture [5] , as pores of a range of sizes greater in effective diameter (~10 nm) than that of the proposed tesserae (~1 nm) are clearly visible ( Fig. 1h ). Some tessera-sized pores might be present in the network, but there are many much larger pores; hence, the tessera model cannot be generally applied. Bands that appear light at lower resolutions contain smaller pores, and may well contain pores smaller than the AFM limit of detection; darker bands contain larger pores. Features were visible both in ambient conditions and under aqueous solution. The observed pores would likely be longitudinally extended, relative to the cell in vivo , due to turgor pressure. Our new in situ AFM imaging method avoided drying or staining artefacts; AFM requires no staining and image features were unaffected by whether the sample was dried during preparation ( Supplementary Fig. S1c,d ). 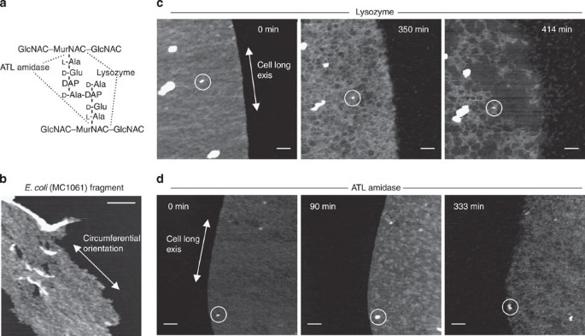Figure 2: Disruption of peptidoglycan architecture visualized by AFM. (a) Targets for lysozyme and ATL amidase. (b) Sacculus fragment from a sample broken by the French press imaged under water, showing persistence of banding outwith the geometrical constraints of cell shape (scale bar, 50 nm; height, 4 nm). (c)In situlysozyme digestion of sacculus under buffer A (scale bar, 100 nm; height, 10 nm). Trapped cytoplasmic material is resistant to the enzyme and acted as a fiduciary marker (circles). (d)In situATL amidase digest of sacculus under buffer A (scale bar, 100 nm; height 10 nm). Figure 2: Disruption of peptidoglycan architecture visualized by AFM. ( a ) Targets for lysozyme and ATL amidase. ( b ) Sacculus fragment from a sample broken by the French press imaged under water, showing persistence of banding outwith the geometrical constraints of cell shape (scale bar, 50 nm; height, 4 nm). ( c ) In situ lysozyme digestion of sacculus under buffer A (scale bar, 100 nm; height, 10 nm). Trapped cytoplasmic material is resistant to the enzyme and acted as a fiduciary marker (circles). ( d ) In situ ATL amidase digest of sacculus under buffer A (scale bar, 100 nm; height 10 nm). Full size image Our imaging showed that circumferential organization was only present at relatively large scale. Nano-dissection using peptidoglycan hydrolases allowed investigation of the contribution of glycan–glycan and glycan–peptide bonds in architecture ( Fig. 2b–d and Supplementary Movies S2,3 ). Digestion with lysozyme, which targets the glycan–glycan bonds, led to the formation of increasingly large pores in the “filigree” until it was completely solubilized. This suggests glycans running planar to the cell membrane but without circumferential orientation. Digestion with Atl amidase [23] , which cuts the glycan–peptide bonds, led to bunching of material into raised knobbles before complete solubilization. Amidase digestion removes peptides leaving only glycans, and would have been expected to reveal a general glycan strand orientation, had there been one. Instead, there is apparent bunching of material. This may be due to the peptidoglycan polymers adopting a relaxed confirmation, potentially indicating that some parts of the network remained under tension even after turgor was removed and contracted in response to hydrolysis of bonds. A French press forces cells through a small aperture under pressure, causing them to break open, freeing cytoplasmic contents. Imaging sacculi from cells broken by the French press ( Fig. 2a and Supplementary Fig. S1l ) revealed fragments of material similar in overall shape to those seen by TEM [24] . The architecture was the same as sacculi from intact cells with no discernible difference between the inside and outside; thus, bands and “filigree” are not dependent on geometrical constraints of overall sacculus shape. Sacculi broke circumferentially, along the short axis, attributable to porous bands where fewer bonds are present ( Supplementary Fig. S1l ). Gram-negative sacculi are more elastic longitudinally than circumferentially: an elastic anisotropy [21] . Glycans are expected to have a higher spring constant than peptides [7] , [21] . If glycans were circumferentially oriented, the anisotropy would have been accounted for by circumferential orientation of less-elastic glycans and consequential longitudinal orientation of more elastic peptides. However, based on our observations, the anisotropy would be better attributed to the orientation of the circumferential bands where more material is present, which would be less elastic than the intervening regions. Thus, the best current explanation is that in vivo circumferential stress on the peptidoglycan is borne by architectural features containing more material. We have determined that E. coli peptidoglycan has a previously unconceived tier of organization in the form of circumferential bands. These are made up of a “filigree” network of features, which becomes increasingly porous on enzymatic digestion, suggesting glycans have no general orientation and are generally planar to the cell surface. As the peptidoglycan has a novel banding architecture with regions of differential porosity, to explain biosynthesis we need to determine the insertion pattern of nascent material to formulate a compatible growth model. Peptidoglycan insertion pattern Fluorescent vancomycin can be used to label sites of peptidoglycan incorporation in Gram-positive bacteria, as it targets the D-ala-D-ala motif associated with unmodified and therefore nascent material [8] , [9] . Vancomycin can also be detected by immunofluoresence when bound to E. coli sacculi [13] . The outer membrane generally prevents vancomycin from reaching the periplasm of the Gram-negative bacteria, but we were able to develop a method to fix and treat E. coli cells so as to allow vancomycin binding to occur (Methods). We then established a means of directly labelling sacculi with fluorescent vancomycin to provide further evidence of the specificity of binding. Fluorescence microscopy revealed distinct regions of synthesis associated with division septa, where one would expect a lot of peptidoglycan insertion would take place ( Fig. 3a–d ). This was apparent regardless of whether cells or sacculi were the subject of labelling, and was common to E. coli (MC1061, MG1655 and MG1655 Δ dacA [25] ) and Caulobacter crescentus (NA1000). Increased labelling was seen in the E. coli (MG1655 Δ dacA ) mutant (known to have increased numbers of D-ala-D-ala motifs). It is surprising that there was labelling of cell poles, as these are known to contain large amounts of relatively old material, which is not partitioned during growth [12] ; growth does not occur at the poles. However, this does not preclude the presence of the D-ala-D-ala motifs introduced by remodelling of peptidoglycan. Deconvolved images of cells seem to show variously sized swathes of labelled material all along the cell cylinder, with no overriding orientation ( Fig. 3a ). However, the resolution of standard fluorescence microscopy does not allow accurate assessment of nascent peptidoglycan insertion. Thus, we constructed a STORM [19] , [20] to resolve the nanoscale insertion pattern. Our system is capable of ~40 nm resolution (Methods) and shows that there are multiple distinct foci of nascent peptidoglycan insertion, from single motifs through to ~50 nm clusters ( Fig. 3e-f ). As a final confirmation of our observations and the specificity of labelling, we labelled sacculi from broken cells ( Supplementary Fig. S2 ) and were thereby able to exclude any potential for non-specific labelling of trapped cytoplasmic contents (known to be present in some intact sacculi, but absent from sacculus fragments, from our AFM imaging). 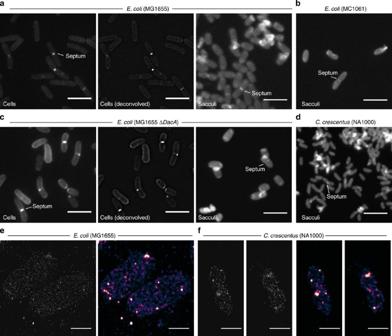Figure 3: Peptidoglycan insertion visualized by fluorescent vancomycin labelling. (a)E. coli(MG1655) cells showing septal labelling, deconvolved cells showing apparently discontinuous labelling of the cylindrical part of the cell wall and sacculi, demonstrating specificity of labelling. (b)E. coli(MC1061) sacculi, similar to those ofE. coli(MG1655). (c)E. coli(MG1655 ΔdacA) cells showing characteristic morphological defects compared with wild type, and increased level of labelling, deconvolved cells (showing apparently discontinuous labelling) and sacculi. (d)C. crescentus(NA1000) sacculi showing similar labelling pattern toE. coli. (f) STORM images ofE. coli(MG1655) sacculi showing foci of insertion. (e) STORM images ofC. crescentus(NA1000) sacculi showing a similar pattern of foci withE. coli(MG1655); (a–d) Scale bars, 5 μm; (e,f) scale bars, 1 μm. Figure 3: Peptidoglycan insertion visualized by fluorescent vancomycin labelling. ( a ) E. coli (MG1655) cells showing septal labelling, deconvolved cells showing apparently discontinuous labelling of the cylindrical part of the cell wall and sacculi, demonstrating specificity of labelling. ( b ) E. coli (MC1061) sacculi, similar to those of E. coli (MG1655). ( c ) E. coli (MG1655 Δ dacA ) cells showing characteristic morphological defects compared with wild type, and increased level of labelling, deconvolved cells (showing apparently discontinuous labelling) and sacculi. ( d ) C. crescentus (NA1000) sacculi showing similar labelling pattern to E. coli . ( f ) STORM images of E. coli (MG1655) sacculi showing foci of insertion. ( e ) STORM images of C. crescentus (NA1000) sacculi showing a similar pattern of foci with E. coli (MG1655); ( a – d ) Scale bars, 5 μm; ( e , f ) scale bars, 1 μm. Full size image Peptidoglycan insertion in Gram-negative bacteria occurs in multiple distinct foci spread over the cylindrical portion of the cell. This is surprising, as the elongation machinery moves about the cell in a helical manner [15] , and it is often assumed that peptidoglycan insertion would follow this helical pattern. However, Lpo proteins, required for peptidoglycan synthesis, are present in patches all over the cell [16] , [17] . There must be additional factors acting to guide insertion. Conservation of peptidoglycan architecture in Gram-negative bacteria To determine the level of conservation of peptidoglycan architecture in Gram-negative bacteria, we imaged C. crescentus , Pseudomonas aeruginosa and Campylobacter jejuni sacculi by AFM ( Fig. 4 ). These exhibited a similar architecture to E. coli . Stalks were present in C. crescentus sacculi without banding. In some P. aeruginosa sacculi, multiple large pores (for example, Supplementary Fig. S3b : diameter 13 nm, s.d. 5 nm, n =11) were present near the poles ( Fig. 4c ). This is the location of multiple pili, and the pores could accommodate the 18.5 nm diameter trans-periplasmic type IV secretion systems [26] , one of which is required for each pilus (note that tip convolution generally leads to AFM, underestimating the length measurements at this scale). In some C. jejuni sacculi, one or two large polar pores (>25 nm diameter; Fig. 4h ) were present; these could demark flagellum motor sites [27] . 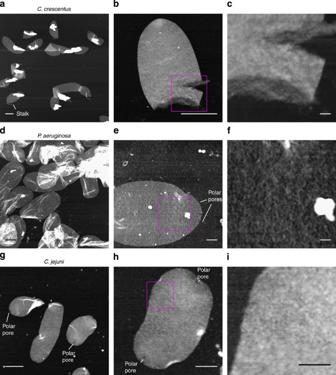Figure 4: AFM images ofC. crescentus,P. aeruginosaandC. jejunisacculi. (a)C. crescentussacculi showing stalks (scale bar, 750 nm; height 20 nm). (b) BrokenC. crescentussacculus (scale bar, 500 nm; height, 7 nm). (c) Close up of boxed region frombshowing “filigree” porous network architecture (scale bar, 50 nm; height, 7 nm). (d) Field ofP. aeruginosasacculi (scale bar, 500 nm; height, 8 nm). (e)P. aeruginosasacculus (scale bar, 200 nm; height, 6 nm). (f) Close up of boxed region incshowing architecture (scale bar, 50 nm; height, 6 nm). (g) Field ofC. jejunisacculi (scale bar, 500 nm; height, 4 nm). (h)C. jejunisacculus (scale bar, 200 nm; height, 4.5 nm). (i) Close up of boxed region fromh, showing disordered “filigree” network (scale bar, 100 nm; height, 3.5 nm). Figure 4: AFM images of C. crescentus , P. aeruginosa and C. jejuni sacculi. ( a ) C. crescentus sacculi showing stalks (scale bar, 750 nm; height 20 nm). ( b ) Broken C. crescentus sacculus (scale bar, 500 nm; height, 7 nm). ( c ) Close up of boxed region from b showing “filigree” porous network architecture (scale bar, 50 nm; height, 7 nm). ( d ) Field of P. aeruginosa sacculi (scale bar, 500 nm; height, 8 nm). ( e ) P. aeruginosa sacculus (scale bar, 200 nm; height, 6 nm). ( f ) Close up of boxed region in c showing architecture (scale bar, 50 nm; height, 6 nm). ( g ) Field of C. jejuni sacculi (scale bar, 500 nm; height, 4 nm). ( h ) C. jejuni sacculus (scale bar, 200 nm; height, 4.5 nm). ( i ) Close up of boxed region from h , showing disordered “filigree” network (scale bar, 100 nm; height, 3.5 nm). Full size image The architecture in all Gram-negative species, the sacculi of which we visualized by AFM, was essentially similar. Our observed peptidoglycan architecture and insertion pattern do not fit with existing models for cell wall structure and dynamics. The most plausible explanation for the data is that certain regions of the sacculi are more permissive for peptidoglycan insertion than others. It is unlikely that these would be areas where there is a lot of pre-existing peptidoglycan, as that would lead to those regions becoming interminably denser and thicker, with no potential for growth. We therefore propose a new peptidoglycan-architecture-regulated model of growth where insertion of peptidoglycan takes place only in the regions of the sacculus with the most and largest pores ( Fig. 5 ). If these regions have a permissive architecture, negative feedback would act, as they acquire more material during biosynthesis leading to a non-permissive architecture. The peptidoglycan biosynthetic apparatus includes penicillin binding proteins (PBPs), and is mediated by mobile [15] , cytoskeletal [28] , [29] , MreB, which gives it an overall circumferential orientation. Biosynthesis also requires the outer membrane protein LpoA [16] , [17] , which has to span the peptidoglycan layer and interact with PBP1A to permit the incorporation of new material. The interaction, and hence biosynthesis, can only occur in the more porous regions of the peptidoglycan and is inhibited by deposition of new material, thus providing a regulatory mechanism for control of peptidoglycan thickness and location of synthesis. Growth can then occur as the non-permissive, less porous regions are ultimately hydrolysed and stretched under turgor, leading to cell elongation, and once again becoming permissive for insertion. There are multiple peptidoglycan hydrolases in E. coli [30] , some forming complexes with PBPs [3] , suggesting spatio-temporal linkage of peptidoglycan metabolism, compatible with our architecture-regulated model of insertion. 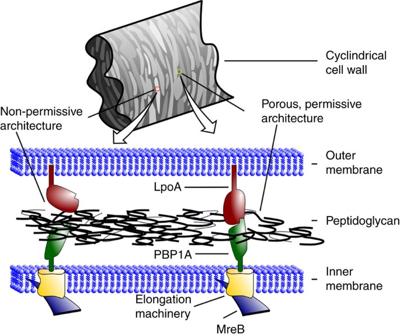Figure 5: Model of peptidoglycan insertion based on AFM, fluorescence microscopy and STORM data. Regions of porous architecture (dark bands in AFM images) are permissive for insertion of new peptidoglycan, which occurs when the elongation machinery is present, and PBP1A and LpoA are able to form a complex, resulting in the patchy pattern of insertion illustrated by STORM images. Figure 5: Model of peptidoglycan insertion based on AFM, fluorescence microscopy and STORM data. Regions of porous architecture (dark bands in AFM images) are permissive for insertion of new peptidoglycan, which occurs when the elongation machinery is present, and PBP1A and LpoA are able to form a complex, resulting in the patchy pattern of insertion illustrated by STORM images. Full size image Gram-negative peptidoglycan is more disordered than previously thought [4] ; the peptidoglycan layer is a porous three-dimensional polymer network with differentiated bands. This architecture, in concert with the spatial ordering components of the elongation machinery, enables high-fidelity propagation of cell shape and cell wall thickness, resulting in a new model of architecture and synthesis, applicable to several Gram-negative species. The next challenges will be to elucidate the roles of individual synthetic and autolytic enzymes in the generation of the architecture we have observed, and to associate architectural complexity with the chemical diversity apparent from muropeptide analyses. Purification of peptidoglycan Peptidoglycan was purified using a standard procedure for Gram-negative organisms (see Supplementary Table S1 for strains and growth conditions). Cells were grown to exponential phase (optical density (OD) 600 ~0.3) or stationary phase (OD 600 ~1), chilled on ice, collected by centrifugation (8,000 g , 10 min) and resuspended in PBS at 4 °C. Where stated, samples were broken by the French press at 4 °C. Breakage was confirmed by optical microscopy. The PBS suspension was then added dropwise to boiling 5% w/v SDS in distilled water. The resulting mixture was then boiled for 30 min and washed three times by ultracentrifugation (400 000 g for 15 min at room temperature). This was resuspended in sodium phosphate buffer (50 mM, pH 7.3) containing 100 μg ml −1 α-chymotrypsin and 0.05% w/v sodium azide, and incubated overnight at 37 °C, with agitation at 250 r.p.m. Material was collected by ultracentrifugation then resuspended in 5% w/v SDS and boiled for 30 min. The resulting suspension was washed twice by ultracentrifugation as before, and then resuspended in HPLC grade water, aliquoted and flash frozen with liquid nitrogen. In exception to this method, E. coli (BL21 and W3110) and C. crescentus cells were added directly to SDS before boiling. There was no apparent difference between this method, SDS treatment and that described above. Further purification was as above. Preparation of AFM samples Aliquots of sacculi were defrosted at 4 °C, diluted in 5 mM HCl and incubated at room temperature for 10 min, to aid dispersal of sacculi. C. crescentus sacculi were placed in an ultrasonic bath for 20 min to aid dispersal; this did not interfere with sacculus architecture. A 10-μl drop was applied to freshly cleaved mica, dried with flowing nitrogen, then washed three times with HPLC grade water before further nitrogen drying. Preparation of AFM samples without drying Aliquots were defrosted at 4 °C then diluted in sodium citrate/citric acid buffer (10 mM, pH 3) and incubated at room temperature for 10 min. In parallel with this incubation, 50 μl of nickel chloride (15 mM in 5 mM HCl) was applied to freshly cleaved mica and incubated for 10 min. The nickel–mica was washed three times with HPLC grade water and dried with nitrogen. Then, 50 μl of sacculus suspension was applied to the nickel–mica and incubated for 1 h, and subsequently washed three times with HPLC grade water and transferred to the AFM without being allowed to dry. Preparation of AFM samples for mechanical stretching (“The Rack”) A large glass coverslip was glued to a glass slide to provide a flat substrate. Polydimethylsiloxane (PDMS, QSil 216, ACC Silicones) was prepared by mixing the polymer 10:1 w/w with the cross-linker, then degassing using a vacuum pump to avoid bubbles. The liquid PDMS was then cast against the coverslip by baking at 60 °C for at least 2 h. The resulting sheet of PDMS (~2 mm thick) was cut into a dogbone shape with a razorblade so as to fit the stretching apparatus. A 21 μg ml −1 Cell Tack solution [31] was prepared in sodium bicarbonate buffer (100 mM, pH 8.3). Then, 30 μl of the solution was pipetted onto the PDMS and incubated for 15 min before being washed 15 times with HPLC grade water. Without allowing the surface to fully dry, 10 μl of sacculus suspension in 1 mM HCl was added and the surface subsequently dried with nitrogen. AFM imaging AFM imaging was carried out using a Multimode AFM with extended Nanoscope III controller, apart from the mechanical stretching experiments that were conducted on a Dimension AFM with Nanoscope IV controller. All imaging was carried out in tapping mode. Silicon cantilevers (Olympus AC160TS) were used for imaging in ambient conditions. Silicon nitride cantilevers with silicon tips (Bruker SNL, k~0.32 Nm −1 ) were used for imaging in liquid. For thickness measurements, the AFM was calibrated using silicon atomic steps (NT-MDT, STEPP). AFM image processing, including a three-dimensional display of data, was carried out using Gwyddion (version 2 or later). Pore-size measurements Two roughly orthogonal measurements were taken and averaged for each pore. Sample roughness precluded use of thresholding measurements. In situ enzyme digests Samples were prepared as described above, loaded into the AFM and allowed to equilibrate for several hours under “Buffer A” (10 mM Tris HCl, 1 mM calcium chloride, pH 7.5), then imaged. Enzymes were added (to 10 μg ml −1 ) to the fluid cell by exchanging buffer A for the same, but containing the enzyme of interest. This was done with the tip retracted using the z-piezo. Several exchanges of buffer containing enzyme were carried out in the course of the experiments to counter reduction in buffer volume owing to evaporation. Mechanical stretching A home-built stretching apparatus (“The Rack”) was constructed comprising two opposing stepper motors mounted with clamps to allow pulling on a piece of elastic material about 30 mm in length. These were controlled using Labview software such that strain could be applied incrementally. This device was mounted on a Dimension AFM for imaging the elastic material. Sacculi were prepared on elastic PDMS and imaged between incremental applications of strain. Labelling of E. coli with fluorescent vancomycin All growth took place at 37 °C with agitation. Cultures were grown overnight in lysogeny broth and used to inoculate subsequent cultures to OD 600 =0.05. These were allowed to grow to OD 600 ~0.3 to 0.4 (exponential phase). Cells were fixed by adding 5 ml culture to 5 ml fixing solution (4 ml PBS+1 ml 16% w/v paraformaldehyde) and incubated on a rotary shaker for 15 min at room temperature. Cells were collected by centrifugation (5,000 g , 10 min) and pellets resuspended in 1 ml PBS before being washed twice by centrifugation (14,000 g , 1 min). Cells were then incubated in 1 ml 0.1% v/v Triton X-100, 5 mM EDTA in PBS for 45 min at room temperature before being washed three times in PBS as before. Cells were resuspended in 1 ml PBS to which fluorescent vancomycin (prepared using a succinimidyl ester of Alexa Fluor 532 (Invitrogen, A-20001) as previously described [8] ) was added to a final concentration of 4 μg ml −1 . The sample was protected from light and incubated at room temperature for 5 min before being washed by centrifugation (14,000 g , 1 min) with water. Cells were resuspended in water and deposited on an agarose pad or poly-l-lysine coated slide for imaging. Labelling of sacculi with fluorescent vancomycin Coverslips were sonicated for 15 min in 1 M KOH, washed with copious water and dried with nitrogen [32] . If intended for super-resolution microscopy, coverslips were sparsely coated with fiducial 103 nm diameter gold nanoparticles (Nanopartz, 13-100-25). Sacculi were then deposited onto coverslips as described for AFM on mica. The sacculi were labelled by applying a 50 μl drop of 4 μg ml −1 fluorescent vancomycin in water and incubating for 15 min, before thoroughly washing with water and drying with nitrogen. The coverslips were mounted on the slides before imaging with either 5 μl Slow Fade Gold (Invitrogen, S36936) for deconvolution microscopy or 5 μl PBS containing 10 mM cysteamine for super-resolution microscopy. Deconvolution microscopy Deconvolution microscopy was conducted as previously described [10] . Images were processed in ImageJ (version 1.45g). Super-resolution microscopy Direct STORM imaging was used [33] . A 100-mW, 532-nm diode laser (Laser 2000) was focussed onto the back plane of a 60 × , numerical aperture 1.4 oil immersion objective mounted in an Olympus IX71 inverted optical microscope. A filter cube containing a 552-nm longpass dichroic filter (Semrock FF552-DI02) and a 565(24)-nm bandpass emission filter (Semrock Brightline 565/24) was inserted for STORM. A piezoelectric motor (Physik Instrumente) was used to adjust focus. An image expander comprising a 35-mm and a 100-mm lens was used to project the image onto a Hamamatsu ImagEM camera set to acquire at 50 frames per second. A 1-m focal length cylindrical lens was inserted between the image expander lenses to allow for compensation of drift perpendicular to the focal plane [32] . Focus was maintained by repeatedly localizing a fiducial particle and adjusting the lens position using the piezo to maintain the ratio of the fitted full-width half maxima (FWHM) in perpendicular directions at 1:1. Laser power was adjusted by pulse-width modulation to maximize signal without saturating the charge-coupled device. The camera and piezo were controlled using Labview (version 10). Image processing was conducted using photoactivation localization microscopy/STORM methodology as previously described by others [19] , [32] . Data were processed by fitting Gaussian functions to individual molecule fluorescence, identified by very clear intrinsic blinks, using Matlab. Drift in the focal plane was corrected retrospectively by tracking a fiducial particle throughout the acquisition sequence and offsetting localizations against its position. Super-resolution images were rendered by creating an image of desired pixel size and marking each pixel to which a blink event was localized bright. A 30-nm Gaussian blur was applied in ImageJ (version 1.46c). Resolution can be estimated by taking the FWHM of position distributions for molecules that emit light in five or more sequential frames, providing an estimate of error pertinent to a dye molecule. For example, this resulted in FWHM x ~42 nm and FWHM y ~44 nm for the image in Fig. 3e , and FWHM x ~35 nm, FWHM y ~34 nm for the image in Fig. 3f . Resolution was not estimated using fiducial particles, as these were much brighter than the dye molecules under the imaging conditions employed, and would therefore make resolution appear artificially better than it was. How to cite this article: Turner, R.D. et al . Cell wall elongation mode in Gram-negative bacteria is determined by peptidoglycan architecture. Nat. Commun. 4:1496 doi: 10.1038/ncomms2503 (2013).